Age-related variations in the methylome associated with gene expression in human monocytes and T cells Age-related variations in DNA methylation have been reported; however, the functional relevance of these differentially methylated sites (age-dMS) are unclear. Here we report potentially functional age-dMS, defined as age- and cis -gene expression-associated methylation sites (age-eMS), identified by integrating genome-wide CpG methylation and gene expression profiles collected ex vivo from circulating T cells (227 CD4+ samples) and monocytes (1,264 CD14+ samples, age range: 55–94 years). None of the age-eMS detected in 227 T-cell samples are detectable in 1,264 monocyte samples, in contrast to the majority of age-dMS detected in T cells that replicated in monocytes. Age-eMS tend to be hypomethylated with older age, located in predicted enhancers and preferentially linked to expression of antigen processing and presentation genes. These results identify and characterize potentially functional age-related methylation in human T cells and monocytes, and provide novel insights into the role age-dMS may have in the aging process. Advancing age is associated with extensive changes in human physiology, and is the most important risk factor for many diseases. Age-related changes in gene expression are thought to underlie many of these physiologic and pathologic consequences of aging [1] . To better understand age-related changes in gene expression, it is important to consider changes in mechanisms that regulate gene expression, such as epigenetic modifications including DNA methylation of cytosines in CpG dinucleotides and histone modifications [2] , [3] . Previously, we investigated differentially methylated CpG sites (dMS) in 1,264 CD14+ monocyte samples for potential functional relationships with cis -gene (±1 Mb) expression [4] , and uncovered many significant (false discovery rate (FDR) <0.001) gene expression-associated methylation sites (eMS). Some of these eMS were very strongly correlated with cis -gene expression, such as CpG site cg17005068. Located in the glutathione S-transferase theta 1 ( GSTT1 ) promoter, methylation of cg17005068 was highly correlated with GSTT1 expression (partial correlation ( prho )=−0.86, P <2.2 × 10 −308 ), and in combination with 15 other GSTT1 -eMS, methylation accounted for 77% of the variance of GSTT1 expression in monocytes [4] . Other recent studies have identified dMS associated with age (age-dMS), including regions with decreased (hypo age-dMS) and increased (hyper age-dMS) methylation with older age [5] , [6] , [7] , [8] , [9] , [10] . However, the results from previous studies investigating the relationships between age-dMS and gene expression are inconclusive [11] , [12] , [13] , [14] , [15] . One of the most comprehensive studies measured methylation and gene expression in the whole blood of 168 individuals, and reported significant negative correlations between age-dMS and gene expression [12] , while another study measuring methylation and gene expression in different samples reported negligible relationships between age-dMS and gene expression [15] . Small sample sizes, mixed cell samples, and gene expression and methylation data measured in different samples makes findings from previous studies difficult to interpret. Overall, there is still a lack of clear understanding of the effects of age-dMS on the transcriptome [16] . 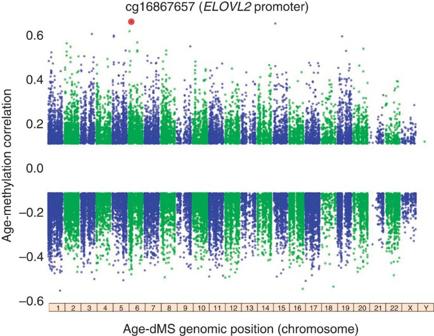Figure 1: The aging methylome in 1,264 monocyte samples. The analysis of age and methylation in 1,264 CD14+ monocyte samples included 448,523 CpG sites, of which 37,911 had methylation associated with age (age-dMS; 26,159 negatively associated, 11,752 positively associated, FDR<0.001). The most significant age-dMS (red circle, cg16867657,prho=0.66, FDR=3.65 × 10−140) was detected on chromosome 6 in the ELOVL fatty acid elongase 2 (ELOVL2) promoter. The partial correlation between CpG methylation and age is shown ony-axis, compared with CpG genomic location (by chromosome,x-axis). Linear regression analysis also included the following covariates: race, sex, site of data collection, microarray chip and residual sample contamination with non-targeted cells (see Methods). To better understand the functional implications of age-dMS, and to identify age-dMS that potentially mediate the relationship between age and gene expression, here we utilized methylomic and transcriptomic data from 1,264 CD14+ purified monocyte samples, collected from a large population of community-dwelling participants in the Multi-Ethnic Study of Atherosclerosis (MESA), ranging in age from 55 to 94 years ( Supplementary Table 1 ), as well as methylomic and transcriptomic data from 227 CD4+ T cell samples from a subset of the population. We identified, cross-sectionally, potentially functional age-associated methylation signals that were correlated with cis -gene expression and clinical measures of vascular aging (pulse pressure eMS), and provide detailed functional annotation from publicly available datasets (for example, ENCODE) characterizing the genomic landscape surrounding these potentially functional methylation sites. Identification of age-dMS We first characterized DNA methylation at ~450,000 CpG sites across the genome in CD14+ purified cells (predominately monocytes) and CD4+ purified cells (T cells) collected from 227 MESA individuals. Using association analysis with a FDR threshold of 0.001, and adjusting for biological and technical covariates (Methods), we identified 2,285 monocyte-specific age-dMS, 2,023 T-cell-specific age-dMS, and 572 overlapping age-dMS across the two cell types. We then expanded our monocyte sample size to 1,264 MESA individuals, and identified 37,911 CpG sites with age-associated methylation (~8% of all CpG sites, FDR<0.001; Fig. 1 ). The majority of age-dMS we detected in 227 T-cell samples shared a similar effect direction between methylation and age as detected in the 1,264 monocyte samples ( Supplementary Fig. 1a and Supplementary Data 1 ). Many of the most significant age-dMS detected in both monocytes and T cells were previously reported to have age-associated methylation measured in whole blood [17] , including CpG sites in ELOVL2 (ELOVL fatty acid elongase 2; cg16867657, prho =0.66, FDR=3.65 × 10 −140 ), FHL2 (four and a half LIM domains 2; cg06639320, prho =0.55, FDR=4.45 × 10 −88 ) and PENK (proenkephalin; cg16419235, prho =0.52, FDR=2.85 × 10 −75 ). Figure 1: The aging methylome in 1,264 monocyte samples. The analysis of age and methylation in 1,264 CD14+ monocyte samples included 448,523 CpG sites, of which 37,911 had methylation associated with age (age-dMS; 26,159 negatively associated, 11,752 positively associated, FDR<0.001). The most significant age-dMS (red circle, cg16867657, prho =0.66, FDR=3.65 × 10 −140 ) was detected on chromosome 6 in the ELOVL fatty acid elongase 2 ( ELOVL2 ) promoter. The partial correlation between CpG methylation and age is shown on y -axis, compared with CpG genomic location (by chromosome, x -axis). Linear regression analysis also included the following covariates: race, sex, site of data collection, microarray chip and residual sample contamination with non-targeted cells (see Methods). Full size image Characterization of hyper and hypo age-dMS We next examined the enrichment of 37,911 monocyte age-dMS from our 1,264 monocyte samples, within genomic regions with predicted roles in regulating gene expression (for example, enhancers) based on histone modifications, CCCTC-binding factor (CTCF) binding and DNase hypersensitivity reported in a monocyte sample by ENCODE [18] , [19] . Age-dMS exhibiting increased methylation with age (hyper age-dMS) were located in distinctly different functional domains than age-dMS exhibiting decreased methylation with age (hypo age-dMS), consistent with previous reports [6] , [10] , [20] . Compared to all CpG sites tested, hyper age-dMS were significantly enriched for inactive/repressive histone modifications [18] (H3K27me3, bivalent H3K27me3/H3K4me3), while being depleted for active chromatin marks [3] , [18] , [21] (H3K4me3, H3K27ac ( Fig. 2a ). However, there was no clear preference for hypo age-dMS among inactive versus active histone modifications (fold enrichments ranging: 0.9–1.1). We also replicated previous findings [10] , [14] , [22] that hyper age-dMS are enriched among CpG islands ( Fig. 2b ) and 1st exons ( Fig. 2c ), while hypo age-dMS are enriched among CpG island ‘shores’, and the 3′ untranslated regions of genes. 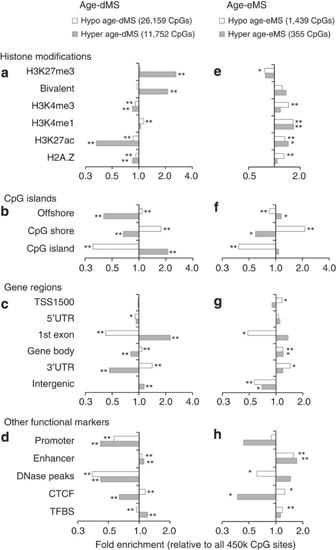Figure 2: Enrichment of Age-dMS and Age-eMS in monocytes for regulatory features. Fold enrichment of age-associated CpG sites (37,911 age-dMS, FDR<0.001, left), and fold enrichment of age andcis-gene expression-associated methylation sites (FDR<0.001, 1,794 age-eMS, right), stratified by methylation positively associated with age (hyper age-dMS, shaded) and negatively associated with age (hypo age-dMS, white) for (a,e) histone modifications reported by ENCODE in a monocyte sample, (b,f) CpG islands and ‘shores’, (c,g) gene regions, including: within 1.5 kb upstream of the transcription start site (TSS1500), the 5′ untranslated region (5′ UTR), the 1st gene exon, the gene body, the 3′ UTR or intergenic, and (d,h) predicted gene expression regulatory regions based on histone modifications (enhancer and promoter based on H3K4me1/3, H3K27ac), CTCF binding and DNase peaks reported in a monocyte sample (ENCODE/UCSC browser), and transcription factor binding sites (TFBS) reported in any cell type available from the UCSC Genome Browser. Fold enrichments presented are from 1,264 monocyte samples, and are relative to all 448,523 CpG sites tested (y-axis); *1 × 10−6≤P<0.01, **P<1 × 10−6,χ2-test. Figure 2: Enrichment of Age-dMS and Age-eMS in monocytes for regulatory features. Fold enrichment of age-associated CpG sites (37,911 age-dMS, FDR<0.001, left), and fold enrichment of age and cis -gene expression-associated methylation sites (FDR<0.001, 1,794 age-eMS, right), stratified by methylation positively associated with age (hyper age-dMS, shaded) and negatively associated with age (hypo age-dMS, white) for ( a , e ) histone modifications reported by ENCODE in a monocyte sample, ( b , f ) CpG islands and ‘shores’, ( c , g ) gene regions, including: within 1.5 kb upstream of the transcription start site (TSS1500), the 5′ untranslated region (5′ UTR), the 1st gene exon, the gene body, the 3′ UTR or intergenic, and ( d , h ) predicted gene expression regulatory regions based on histone modifications (enhancer and promoter based on H3K4me1/3, H3K27ac), CTCF binding and DNase peaks reported in a monocyte sample (ENCODE/UCSC browser), and transcription factor binding sites (TFBS) reported in any cell type available from the UCSC Genome Browser. Fold enrichments presented are from 1,264 monocyte samples, and are relative to all 448,523 CpG sites tested ( y -axis); *1 × 10 −6 ≤ P <0.01, ** P <1 × 10 −6 , χ 2 -test. Full size image Histone modifications (H3K4me1/3 and H3K27ac), CTCF binding and DNase peaks previously reported in a monocyte (CD14+) sample [19] were also used to predict monocyte-specific functional regions, including promoters, enhancers and insulators. Both hyper and hypo age-dMS were depleted among predicted promoter regions and DNase peaks, while being enriched among enhancer regions ( Fig. 2d ). Hypo age-dMS were also enriched for CTCF binding sites; however, hyper age-dMS were not. We also report the enrichment of age-dMS among transcription factor binding sites (TFBS) reported in any cell type available from the UCSC Genome Browser [23] (due to the lack of monocyte-specific TFBS). Hyper age-dMS showed some enrichment among these sites, while hypo age-dMS did not. Identification of age-eMS Potentially functional age-dMS were defined as CpG sites whose % methylation was associated with age (FDR<0.001) and with mRNA expression of any gene within 1 Mb of the CpG site in question (FDR<0.001). Among 227 T-cell samples, 44 age-dMS were also cis -gene expression-associated methylation sites (age-eMS) (2% of the 2,595 T-cell age-dMS), with methylation correlated with age ( prho ranging:−0.54–0.70) and with cis -gene expression ( prho ranging:−0.62–0.56). Half of these T cell age-eMS (22 CpG sites) had methylation profiles associated with age in 1,264 monocyte samples; however, there was no replication of the association between methylation and gene expression for these 22 CpG sites in monocyte samples ( Supplementary Fig. 1b ). Due to the lack of age-eMS detected in both cell types, combined with our larger monocyte sample size and the availability of monocyte-specific histone modification data from ENCODE [19] , we focus the rest of our age-eMS investigations on findings from 1,264 monocyte samples. We detected 1,794 age-eMS among the 1,264 monocyte samples (4.7% of 37,911 monocyte age-dMS; reported in Supplementary Data 2 ), with methylation correlated with age ( prho range: −0.46–0.44; Fig. 3a ) and cis -gene expression ( prho range: −0.69–0.62; Fig. 3b ). The most significant age-dMS identified as an age-eMS ( Fig. 3a ) in monocytes was detected within a predicted enhancer region of the nuclear factor I-A ( NFIA ) gene body ( Fig. 4a ). NFIA is a transcription factor whose expression drives erythropoiesis, while its silencing drives granulopoiesis [24] . Hypomethylation with age of cg10628205 ( prho =−0.46; FDR=1.06 × 10 −58 ; Fig. 4b ) correlated with increased NFIA expression ( prho =−0.16; FDR=1.97 × 10 −5 ; Fig. 4b ). Five nearby CpG sites were also identified as age-eMS linked with NFIA expression. Using multiple regression analysis including all six NFIA age-eMS in the same model, four age-eMS were found to be independently associated with NFIA expression. In total, methylation of these four CpG sites explained 7.5% of the variance of NFIA gene expression. However, some age-dMS identified as age-eMS had stronger correlations between methylation and gene expression ( Fig. 3b and Supplementary Data 2 ). For instance, the strongest correlation detected was between age-dMS cg10628205 (methylation and age prho =−0.15) and expression of vasohibin 1 ( VASH1 , prho =−0.69). This age-eMS is 42 kb upstream of the VASH1 transcription start site (TSS). VASH1 is an angiogenesis inhibitor that has previously been reported to suppress monocyte and macrophage infiltration of the kidney [25] . 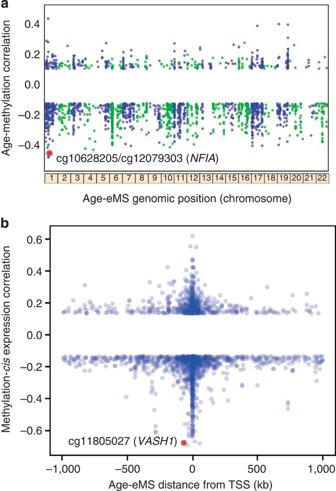Figure 3: Correlations between age-methylation and methylation-gene expression for Age-eMS in 1,264 monocyte samples. CpG sites with methylation associated with age (FDR<0.001) andcis-gene expression (1,794 age-eMS; FDR<0.001;Supplementary Data 2). (a) The partial correlation of age-eMS methylation with age (y-axis), compared with age-eMS genomic location (by chromosome,x-axis); the strongest correlations (prho=−0.46) were between age and methylation of cg10628205 and cg12079303 (red circle), which were also correlated with the expression ofNFIA.(b) The partial correlation between age-eMS methylation andcis-gene expression (y-axis), compared with age-eMS distance to the associated gene transcription start site (TSS,x-axis); the strongest correlation (prho=−0.69) was between methylation of cg11805027 and expression ofVASH1. Linear regression analysis also included the following covariates: race, sex, site of data collection, microarray chip and residual sample contamination with non-targeted cells (see Methods). Figure 3: Correlations between age-methylation and methylation-gene expression for Age-eMS in 1,264 monocyte samples. CpG sites with methylation associated with age (FDR<0.001) and cis -gene expression (1,794 age-eMS; FDR<0.001; Supplementary Data 2 ). ( a ) The partial correlation of age-eMS methylation with age ( y -axis), compared with age-eMS genomic location (by chromosome, x -axis); the strongest correlations ( p rho=−0.46) were between age and methylation of cg10628205 and cg12079303 (red circle), which were also correlated with the expression of NFIA. ( b ) The partial correlation between age-eMS methylation and cis -gene expression ( y -axis), compared with age-eMS distance to the associated gene transcription start site (TSS, x -axis); the strongest correlation ( p rho=−0.69) was between methylation of cg11805027 and expression of VASH1 . Linear regression analysis also included the following covariates: race, sex, site of data collection, microarray chip and residual sample contamination with non-targeted cells (see Methods). 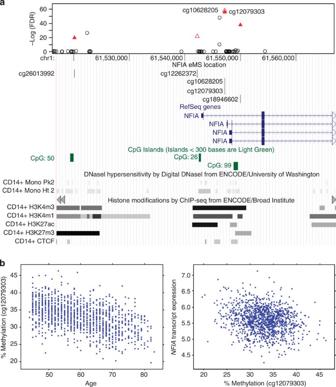Figure 4: Methylation ofNFIAis associated with age and withNFIAexpression in 1,264 monocyte samples. (a) Regional association plot showing the significance (−log10FDR, top panely-axis) of single CpG methylation associations with age surroundingNFIA(nuclear factor I/A) by genomic position on chromosome 1 (x-axis). Six CpG sites nearNFIA(red triangles) have methylation associated with age (FDR ranging from 1.1 × 10−58to 1.2 × 10−16), and with increased expression ofNFIAin monocytes (age-eMS, FDR ranging from 2.0 × 10−11to 3.2 × 10−4). Methylation of four age-eMS have independent effects onNFIAexpression from multiple regression analysis (filled-in triangles, cg00165994 downstream, not shown) with cg12079303 remaining the most significant.NFIAage-eMS overlap histone modification marks indicative of active regulatory regions (that is, H3K4me1/3, H3K27ac by ChIP-seq from ENCODE, bottom panel). (b) cg12079303 methylation is negatively correlated with age (left;prho=−0.46, rho=−0.48) and negatively correlated withNFIAmRNA expression (right;prho=−0.16, rho=−0.12). Full size image Figure 4: Methylation of NFIA is associated with age and with NFIA expression in 1,264 monocyte samples. ( a ) Regional association plot showing the significance (−log 10 FDR, top panel y -axis) of single CpG methylation associations with age surrounding NFIA (nuclear factor I/A) by genomic position on chromosome 1 ( x -axis). Six CpG sites near NFIA (red triangles) have methylation associated with age (FDR ranging from 1.1 × 10 −58 to 1.2 × 10 −16 ), and with increased expression of NFIA in monocytes (age-eMS, FDR ranging from 2.0 × 10 −11 to 3.2 × 10 −4 ). Methylation of four age-eMS have independent effects on NFIA expression from multiple regression analysis (filled-in triangles, cg00165994 downstream, not shown) with cg12079303 remaining the most significant. NFIA age-eMS overlap histone modification marks indicative of active regulatory regions (that is, H3K4me1/3, H3K27ac by ChIP-seq from ENCODE, bottom panel). ( b ) cg12079303 methylation is negatively correlated with age (left; prho =−0.46, rho=−0.48) and negatively correlated with NFIA mRNA expression (right; prho =−0.16, rho=−0.12). Full size image Characterization of hyper and hypo age-eMS The majority of age-eMS were located in close proximity to the associated gene TSS ( Fig. 3b ), with 71% of age-eMS in monocytes located within 100 kb of the TSS. In addition, the correlations between methylation and gene expression of age-eMS located within 100 kb of the TSS tended to be stronger (absolute prho : average=0.22, median 0.18) than age-eMS located further than 100 kb from the TSS ( prho : average=0.17, median=0.16). Age-eMS enriched in open chromatin and enhancer regions In an effort to further explore the potential functionality of the age-eMS identified, we examined the enrichment of age-eMS within genomic regions with predicted roles in regulating gene expression based on histone modifications, CTCF binding and DNase hotspots reported in a monocyte sample by ENCODE [18] , [19] . The most prominent features of age-eMS were their enrichment for histone modifications indicative of open/active chromatin (H3K4me1 and H3K27ac, Fig. 2e ) and predicted enhancer regions ( Fig. 2h ), while being depleted among repressed genomic regions (H3K27me3), for both hypo and hyper age-eMS. Age-eMS linked to antigen processing and presentation genes The presence of predicted functional regions overlapping the identified age-eMS provides additional support for these genomic regions being important regulatory regions. Therefore, we consider age-eMS overlapping enhancers, insulators or promoters (669 age-eMS) as top candidates for potentially functional age-dMS ( Supplementary Data 2 ). These 669 CpG sites overlapping potentially functional regulatory regions are associated with the expression of 403 different genes, which are significantly enriched [26] with antigen processing and presentation genes (Gene Ontology gene set: 0019882, FDR=9.60 × 10 −4 ). Table 1 shows associations between age, methylation and expression of 13 antigen processing and presentation genes including major histocompatibility complex (MHC) class I and II genes. Supporting previous findings [27] , we observe an upregulation of all MHC class I and II genes with expression associated with age (FDR<0.01) ( Supplementary Table 2 ). Table 1 Antigen processing and presentation genes enriched among genes with expression linked to potentially functional age-eMS. Full size table Age-eMS linked with vascular aging To further explore the biological relevance of age-eMS, we identified a subset of 186 age-eMS that were associated with vascular age (FDR<0.001), measured by pulse pressure ( Supplementary Data 2 ). After adjusting for chronological age, 42 age-eMS remained nominally associated with pulse pressure (pulse pressure eMS), some of which were associated with expression of genes that have biologically plausible roles in vascular aging, such as AT rich interactive domain 5B ( ARID5B (MRF1 like)) and gelsolin ( GSN ). ARID5B is a transcription factor that has been implicated in the pathogenesis of coronary artery disease [28] . Gelsolin is an actin binding protein which has been linked to vascular permeability [29] , cell motility and the development of many pathological processes, including cardiovascular diseases [30] . Here we report, for the first time, the relationship between aging, DNA methylation and cis -gene expression at the global level, using two purified cell types from the same individuals in a large cohort study. We find that only a small fraction of dMS (~2%) associated with aging were also associated with differential expression of nearby genes in 227 T-cell samples. In parallel, we saw a slightly larger proportion of age-dMS (~5%) associated with cis -gene expression in a larger sample of monocytes (1,264). However, in contrast to age-dMS, no age-eMS were detected in both cell types. The lack of replication of any T-cell age-eMS within monocytes could reflect a cell-specific nature of age-eMS, demonstrating the importance of using purified cells for methylomic and transcriptomic studies. In addition to their association with cis -gene expression, we also found that age-eMS were enriched in enhancers and active chromatin, and are more likely to be hypo than hypermethylated with older age. Notably, age-associated hypomethylation of an enhancer region of NFIA was the most significant age-dMS with c is -gene expression-associated methylation. Supporting the potential functional nature of these sites, decreased NFIA expression has been linked with increasing methylation of these CpG sites in response to all- trans retinoic acid treatment in a myeloid leukaemia cell line [24] . Our age-dMS results are in agreement with many previous findings. Hyper age-dMS are more likely to occur in CpG islands [5] , [10] , [12] , [13] , [14] and inactive chromatin [6] , [10] , [12] , [13] , [15] , [31] . Conversely, we found hypo age-dMS are more likely to occur in CpG shores and insulator regions [10] , [14] , [15] , [31] . Why are so few age-dMS associated with gene expression? The occurrence of dMS has been proposed to be a highly polymorphic and stochastic process occurring during cell division [32] , yet one that still results in consistent dMS across the genome due to chromatin state and sequence-specific factors (for example, CpG density and TFBS) which may influence the likelihood of differential methylation [33] . Thus, it is plausible that age-dMS may form stochastically as function of cell division (mitotic age), and are allowed to accumulate at specific, permissive locations. However, age-dMS have been reported in post-mitotic tissues [5] , [10] , [15] , and across cells showing a wide range of proliferative capabilities [15] , suggesting mitotic age alone does not explain the occurrence of age-dMS. Indeed, we found substantial overlap between age-dMS identified in two cell types with highly distinct replicative profiles (monocytes and T cells). Whether they occur as a function of mitotic age, or some other age-associated factors, the robust occurrence of age-dMS could be linked to their preference for inactive chromatin states and subsequent unimportance for nearby gene expression, thus allowing them to accumulate without harming cellular function. Further, cumulative effects of multiple age-dMS on cis -gene expression [11] may have also been missed by investigating the relationship between individual CpGs with nearby gene expression. Age-eMS, on the other hand, may have more heterogeneous origins, representing both stochastic events that are allowed to occur and persist after loss of cellular homoeostasis with age (for example, cell-specific changes in histone modification patterns and transcription factor expression and activity), and also compensatory mechanisms by the cell in response to other age-related changes. Supporting the link between age-eMS and biological aging, we found that genes with expression linked to potentially functional age-related methylation sites are enriched with antigen processing and presentation genes (MHC class I and II). Upregulation of MHC class II signalling has been implicated in ‘para-inflammation’ and the development of age-related chronic inflammatory diseases and autoimmune diseases [27] , [34] . Our present work supports previous findings that the MHC class II antigen presentation pathway is upregulated with age [27] , and suggests that methylation-based regulatory mechanisms may contribute to the upregulation of this pathway. In summary, we identified and characterized an important subset of age-related methylation patterns that were associated with cis -gene expression in purified cells. These potentially functional methylation sites, particularly those associated with vascular aging or linked with expression of previously implicated ‘aging genes’, may facilitate the prioritization of biologically relevant age-associated methylation loci for future interrogation. Study population The MESA was designed to investigate the prevalence, correlates and progression of subclinical cardiovascular disease in a population cohort of 6,814 participants. Since its inception in 2000, five clinic visits collected extensive clinical, socio-demographic, lifestyle and behaviour, laboratory, nutrition and medication data [35] . The present analysis is primarily based on analyses of purified monocyte samples from the April 2010 to February 2012 examination of 1,264 randomly selected MESA participants (55–94-year-old, Caucasian (47%), African American (21%) and Hispanic (32%), female (51%)) from four MESA field centres (Baltimore, MD, USA; Forsyth County, NC, USA; New York, NY, USA; and St Paul, MN, USA). T cells were also purified from 225 randomly selected samples which already had purified monocytes. The study protocol was approved by the Institutional Review Boards at Johns Hopkins Medical Institutions, University of Minnesota, Columbia University Medical Center and Wake Forest University Health Sciences. All participants signed informed consent. Power calculation We estimate >80% power to detect age explaining as little as 3.0% of the variance of CpG methylation in monocytes, based on a simple linear regression (alpha=0.05, two-sided test) with a Bonferroni correction to adjust for 448,523 CpG sites tested with age, estimated using QUANTO v1.2 ( N =1,264, average age±s.d.=60.2±9.5; ref. 36 ). In T cells we estimate >80% power to detect age explaining as little as 16% of the variance of CpG methylation in age ( N =227). Purification of monocytes and T cells Centralized training of technicians, standardized protocols and extensive quality control (QC) measures were implemented for collection, on-site processing, and shipment of MESA specimens and routine calibration of equipment. Blood was initially collected in sodium heparin-containing Vacutainer CPT cell separation tubes (Becton Dickinson, Rutherford, NJ, USA) to separate peripheral blood mononuclear cells from other elements within 2 h from blood draw. Subsequently, monocytes and T cells were isolated with anti-CD14 and anti-CD4 monoclonal antibody-coated magnetic beads, respectively, using AutoMACs automated magnetic separation unit (Miltenyi Biotec, Bergisch Gladbach, Germany). Based on flow cytometry analysis of 18 specimens, monocyte samples were consistently >90% pure. T cells were isolated from a subset of our population ( N =227) with anti-CD4 monoclonal antibody-coated magnetic beads, respectively, using AutoMACs automated magnetic separation unit (Miltenyi Biotec). Based on flow cytometry analysis of 18 specimens, T-cell samples were consistently >90% pure. DNA and RNA extraction DNA and RNA were isolated from samples simultaneously using the AllPrep DNA/RNA Mini Kit (Qiagen, Inc., Hilden, Germany). DNA and RNA QC metrics included optical density (OD) measurements, using a NanoDrop spectrophotometer and evaluation of the integrity of 18S and 28S ribosomal RNA using the Agilent 2100 Bioanalyzer with RNA 6000 Nano chips (Agilent Technology, Inc., Santa Clara, CA, USA) following manufacturer’s instructions. RNA with RNA integrity scores >9.0 was used for global expression microarrays. The median of RNA integrity for all the analyzed samples was 9.9. Epigenome-wide methylation quantification The Illumina HumanMethylation450 BeadChip and HiScan reader were used to perform the epigenome-wide methylation analysis. The EZ-96 DNA Methylation Kit (Zymo Research, Orange, CA, USA) was used for bisulphate conversation with 1 μg of input DNA (at 45 μl). Bisulfite-converted DNA (4 μl) was used for DNA methylation assays, following the Illumina Infinium HD Methylation protocol. This consisted of a whole genome amplification step followed by enzymatic end-point fragmentation, precipitation and resuspension. The resuspended samples were hybridized on HumanMethylation 450 BeadChips at 48 °C for 16 h. The individual samples were assigned to the BeadChips and to chip position using the same sampling scheme as that for the expression BeadChips. Global expression quantification The Illumina HumanHT-12 v4 Expression BeadChip and Illumina Bead Array Reader were used to perform the genome-wide expression analysis, following the Illumina expression protocol. The Illumina TotalPrep-96 RNA Amplification Kit (Ambion/Applied Biosystems, Darmstadt, Germany) was used for reverse transcription and amplification with 500 ng of input total RNA (at 11 μl). Biotinylated complementary RNA (700 ng) was hybridized to a BeadChip at 58 °C for 16–17 h. To avoid potential biases due to batch, chip and position effects, a stratified random sampling technique was used to assign individual samples (including five common control sample for the first 480 samples) to specific BeadChips (12 samples/chip) and chip position. QC and pre-processing of microarray data Data pre-processing and QC analyses were performed in R ( http://www.r-project.org/ ) using Bioconductor ( http://www.bioconductor.org/ ) packages. For expression data, data corrected for local background were obtained from Illumina’s proprietary software GenomeStudio. QC analyses and bead-type summarization (average bead signal for each type after outlier removal) were performed using the beadarray package [37] . Detection P -values were computed using the negative controls on the array. The neqc function of the limma [38] package was used to perform a normal-exponential convolution model analysis to estimate non-negative signal, quantile normalization using all probes (gene and control, detected and not detected) and samples, addition of a recommended (small) offset, log 2 transformation and elimination of control probe data from the normalized expression matrix. Multidimensional scaling plots showed the five common control samples were highly clustered together and identified three outlier samples, which were excluded subsequently. Bead-level methylation data were summarized in GenomeStudio. Because the Illumina HumanMethylation450 BeadChip technology employs a two-channel system and uses both Infinium I and II assays; normalization was performed in several steps using the lumi package [39] . We first adjusted for colour bias using ‘smooth quantile normalization’. Next, the data were background adjusted by subtracting the median intensity value of the negative control probes. Last, data were normalized across all samples by standard quantile normalization applied to the bead-type intensities and combined across Infinium I and II assays and both colours. QC measures included checks for sex and race/ethnicity mismatches, and outlier identification by multidimensional scaling plots. The final methylation value for each methylation probe was computed as the M -value, essentially the log ratio of the methylated to the unmethylated intensity [40] . The M -value is well-suited for high-level analyses and can be transformed into the beta-value, an estimate of the per cent methylation of an individual CpG site that ranges from 0 to 1 (thus M is logit(beta-value)). The Illumina HumanMethylation450 BeadChip included probes for 485 K CpG sites. Of these 485 K CpG sites, 448,523 passed the following filters: ‘detected’ methylation levels <90% of MESA samples using a detection P -value cut-off of 0.05, 65 control probes which assay highly polymorphic single nucleotide polymorphisms rather than DNA methylation [41] , or overlap with a repetitive element or region. Pre-processing with global normalization removed large position and chip effects across all probes; however, probe-specific chip effects were found for some CpG sites and gene transcripts, while probe-specific position effects existed for some CpG sites but were ignorable for all gene transcripts. These probe-specific effects were included as covariates in all subsequent analyses. The Illumina HumanHT-12 v4 Expression BeadChip included 48k transcripts. Statistical analyses were limited to probes retained after applying the following filters: non-detectable expression in ≥90% of MESA samples using a detection P -value cut-off of 0.0001, overlap with a repetitive element or region, low variance across the samples (<10th percentile) or putative and/or not well-characterized genes, that is, gene names starting with KIAA, FLJ, HS, Cxorf, MGC or LOC. Association analyses The overall goal of the association analysis was to identify associations, at the genome-wide level, between age and CpG site methylation and transcript expression and CpG site methylation. Association analyses were performed using the linear model function of the Stats package and the stepAIC function of the MASS package in R. To identify gene transcripts or methylation sites associated with age, we fit separate linear regression models with age as a predictor of transcript expression or the M -value for each gene transcript or CpG site, respectively. Covariates were sex, race/ethnicity, study site, expression/methylation chip, methylation position (for age-CpG methylation analyses only) and residual sample contamination with non-targeted cells (for example, non-monocytes, see below). To identify methylation sites associated with gene expression in cis , we fit separate linear regression models with the M -value for each CpG site (adjusted for methylation chip and position effects) as a predictor of transcript expression for any autosomal gene within 1 Mb of the CpG site in question. Covariates were age, sex and race/ethnicity, study site, expression chip and residual sample contamination with non-targeted cells. Sex- and ethnicity-stratified analyses were performed as an internal validation and check of generalizability. To look for potential population stratification, we used EIGENSTRAT [42] to compute principal components (PCs) for each race, based on Affymetrix 6.0 array genotype data [43] , and examined the association between the first five PCs and gene expression, as well as CpG methylation, in race-stratified analyses. Less than 1% of expression transcripts and CpG methylation sites were associated with PCs in the Caucasian and African American populations (FDR<0.05). However, 14.7% of gene expression transcripts and 3.1% of methylation sites in the Hispanic population were associated with the first two PCs (FDR<0.05); therefore, analyses in the Hispanic population were adjusted for the first two PCs. Normality-based P -values were obtained for all tests (they were highly similar to permutation-based P -values and produced essentially the same ranking in a subset of 360 samples). P -values were adjusted for multiple testing using the q -value FDR method [44] , separately for each of the three association analyses. To minimize false-positive results, we used the stringent FDR threshold of 0.001. All the reported FDR was calculated at the epigenome-wide level for the entire gene transcripts or methylation probes that were tested. Although other phenotypic traits are available in MESA, only pulse pressure was tested as an age-associated outcome. Association analyses for individual gene transcripts and pulse pressure were performed using the linear model function in R. We fit separate linear regression models with transcript expression as a predictor of pulse pressure. Covariates included sex, race/ethnicity, study site, expression/methylation chip, methylation position (for age-CpG methylation analyses only) and residual sample contamination. One set of analyses was performed with this set of covariates, and another set of analyses also included age as a covariate. To estimate residual sample contamination for monocyte data analysis, we generated separate enrichment scores for neutrophils, B cells, T cells and natural killer cells. We implemented a Gene Set Enrichment Analysis [45] to calculate the enrichment scores using the gene signature of each blood cell type in the ranked list of expression values for each MESA sample. The cell-type-specific signature genes were selected from previously defined lists [46] and passed the following additional filters: at least fourfold more highly expressed in the targeted cell type than in other cell populations and low expression levels in the targeted cells (here monocytes). To minimize spurious associations due to a few highly influential data points, we calculated Cook’s distance [47] for each data point and repeated the analysis after removing the top four samples with the highest Cook’s distance. We then removed associations whose P -values no longer fell below the FDR-based significance threshold. Functional annotation analysis Histone modifications and CTCF binding reported in a CD14+ sample by ENCODE [48] and TFBS in all available cell types were downloaded from the UCSC Genome Browser [19] . Fold enrichment of CD14+ histone markers (H3K27me3, bivalent (H3K27me3/H3K4me3), H3K4me3, H3K4me1, H3K27ac and H2A.Z) among monocyte age-dMS and age-eMS were reported relative to all 448,523 CpG sites tested. Other predicted functional loci such as promoters, enhancers and insulators were predicted based on proximity to a TSS, as well as the presence of overlapping histone modifications [18] (H3K4me1/3 and H3K27ac) or CTCF binding data available from ENCODE in a CD14+ sample. DAVID Bioinformatics Resources 6.7 (refs 49 , 50 ) was used to examine the enrichment (FDR<0.05) of gene ontology pathways for genes with expression associated (FDR<0.001) with methylation of monocyte age-eMS detected among predicted CD14+ promoter, enhancer and insulator regions, against a background of all monocyte expressed genes (14,619 mRNA transcripts). Accession codes. Microarray data presented in this manuscript have been deposited in the Gene Expression Omnibus (GEO) repository under the accession code GSE56047 . How to cite this article: Reynolds, L. M. et al. Age-related variations in the methylome associated with gene expression in human monocytes and T cells. Nat. Commun. 5:5366 doi: 10.1038/ncomms6366 (2014).